Field-induced density wave in the heavy-fermion compound CeRhIn5 Strong electron correlations lead to a variety of distinct ground states, such as magnetism, charge order or superconductivity. Understanding the competitive or cooperative interplay between neighbouring phases is an outstanding challenge in physics. CeRhIn 5 is a prototypical example of a heavy-fermion superconductor: it orders anti-ferromagnetically below 3.8 K, and moderate hydrostatic pressure suppresses the anti-ferromagnetic order inducing unconventional superconductivity. Here we show evidence for a phase transition to a state akin to a density wave (DW) under high magnetic fields (>27 T) in high-quality single crystal microstructures of CeRhIn 5 . The DW is signalled by a hysteretic anomaly in the in-plane resistivity accompanied by non-linear electrical transport, yet remarkably thermodynamic measurements suggest that the phase transition involves only small portions of the Fermi surface. Such a subtle order might be a common feature among correlated electron systems, reminiscent of the similarly subtle charge DW state in the cuprates. Unconventional superconductivity (SC) often appears in strongly correlated materials on the border of magnetism. These same correlations also produce a variety of competing ground states, which can act as new windows to understanding the physics of these correlated materials. Metals containing Ce often show strong electron correlations due to the proximity of the 4 f state to the Fermi energy, leading to strong coupling with the conduction electrons and a multitude of competing states. Since these states are typically close in energy, phase transitions can be induced by small environmental changes such as magnetic fields or pressure. Thus, they pose ideal candidates to investigate the interplay of various correlated ground states. The heavy-fermion superconductor CeRhIn 5 received significant attention due to its particularly feature-rich phase diagram [1] : the local-moment anti-ferromagnetism (AFM, T N ~3.8 K) is suppressed by moderate pressure and ultimately quenched by a first-order phase transition at P c ~17 kbar in zero magnetic field. Magnetic fluctuations associated with this quantum critical point are thought to induce unconventional SC with a relatively high transition temperature T c max ~2.1 K [2] , similar to the related compounds CeCoIn 5 (refs 3 , 4 , 5 , 6 ) and CeIrIn 5 (ref. 7 ). The main finding of our study is the identification of a previously undetected state akin to a density wave (DW) above a critical field H c ~27 T for fields applied along the c axis (‘DW’, Fig. 1a ). The SC and the DW phases share intriguing similarities: both arise in the vicinity of a quantum critical point bounding the AFM phase, and the transition from the AFM metal into both the DW and the SC states [5] appears to be first order. As charge DWs (CDWs) and spin DWs (SDWs) are mainly observed in low-dimensional electronic systems, the DW in CeRhIn 5 most likely appears due to an instability of a low-dimensional Fermi surface [8] , [9] that coexists with three-dimensional (3D) Fermi surface sheets [10] . 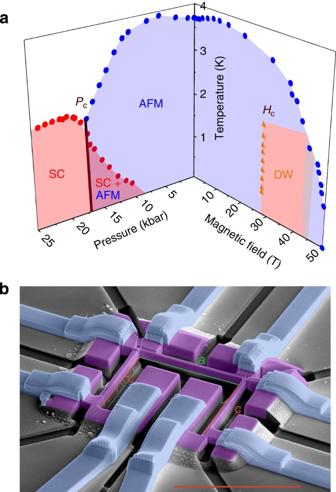Figure 1: Phase diagram of CeRhIn5. (a) Pressure-field phase diagram of CeRhIn5for fields applied along thec-direction. At the critical pressurePc, a first-order phase transition suppressing the anti-ferromagnetism (AFM) occurs within the superconducting state. Under zero applied pressure at the critical magnetic fieldHc, similarly a first-order phase transition into a density wave (DW) state is found, which is the main result of our study. The transition persists up to temperatures of 2 K, above which it becomes unobservable. The DW state clearly coexists with the AFM order, yet it remains an open question if it persists beyond the AFM phase boundary into the paramagnetic state. The (P,T) data is reproduced from ref.35andTN(H) from ref.20. (b) SEM micrograph of a FIB carved ~60 × 60-μm slice of CeRhIn5(purple). Scale bar, 50 μm. The (a,c)-plane-oriented slice was structured into a U-shaped geometry and contacted by FIB-assisted platinum deposition (blue). Through the lower-left contacts, a shared current is applied along the ‘U’, passing through two resistivity bars along thec-direction (red) and one along thea-direction (green). Thecaxis bars are both 31.6 μm long with a cross-section of 1.4 × 4 μm, and theaaxis bar is 34.5 μm long with a cross-section of 2.2 × 4 μm. The high residual resistivity ratios (ρa(300 K)/ρa(80 mK)~258,ρc(300 K)/ρc(80 mK)~268), the good quantitative agreement with the temperature dependence of the resistivity on macroscopic crystals36and the observation of Shubnikov–de Haas oscillations in fields as low as 4 T evidences the high crystal quality of the FIB-prepared devices. Figure 1: Phase diagram of CeRhIn 5 . ( a ) Pressure-field phase diagram of CeRhIn 5 for fields applied along the c -direction. At the critical pressure P c , a first-order phase transition suppressing the anti-ferromagnetism (AFM) occurs within the superconducting state. Under zero applied pressure at the critical magnetic field H c , similarly a first-order phase transition into a density wave (DW) state is found, which is the main result of our study. The transition persists up to temperatures of 2 K, above which it becomes unobservable. The DW state clearly coexists with the AFM order, yet it remains an open question if it persists beyond the AFM phase boundary into the paramagnetic state. The ( P , T ) data is reproduced from ref. 35 and T N (H) from ref. 20 . ( b ) SEM micrograph of a FIB carved ~60 × 60-μm slice of CeRhIn 5 (purple). Scale bar, 50 μm. The ( a,c )-plane-oriented slice was structured into a U-shaped geometry and contacted by FIB-assisted platinum deposition (blue). Through the lower-left contacts, a shared current is applied along the ‘U’, passing through two resistivity bars along the c -direction (red) and one along the a -direction (green). The c axis bars are both 31.6 μm long with a cross-section of 1.4 × 4 μm, and the a axis bar is 34.5 μm long with a cross-section of 2.2 × 4 μm. The high residual resistivity ratios ( ρ a (300 K)/ ρ a (80 mK)~258, ρ c (300 K)/ ρ c (80 mK)~268), the good quantitative agreement with the temperature dependence of the resistivity on macroscopic crystals [36] and the observation of Shubnikov–de Haas oscillations in fields as low as 4 T evidences the high crystal quality of the FIB-prepared devices. Full size image Our observation of DWs in close proximity to unconventional d -wave SC in CeRhIn 5 is reminiscent of the recent developments in the cuprate high- T c superconductors: their particularly complex phase diagram hosts a variety of ground states of correlated electron matter, some coexisting and others competing with high-temperature SC [11] , [12] . One of these states is the spin and charge order, which was initially thought to be a special case for the La-based cuprates such as La 2− x Ba x CuO 4 (refs 12 , 13 ). Yet recently, fluctuating charge order was also observed in YBa 2 Cu 3 O 7− δ (refs 11 , 14 ) and the electronic structure observed by quantum oscillation measurements agrees with the broken translational symmetry due to charge order [15] . Moderate magnetic fields have been observed to influence the charge order, as suggested by X-ray diffraction and nuclear magnetic resonance (NMR) experiments [16] , [17] . While the lattice distortion and the charge modulation may have a profound effect on the electronic structure of the cuprates, by themselves these DWs are subtle features, which could only very recently be identified experimentally. This naturally leads to the question if similarly subtle charge order in the vicinity of unconventional SC is a common feature among several other classes of materials. Our results thus suggest that the coexistence, or competition, between charger order and unconventional SC might be a more common feature among strongly correlated systems than previously thought. Resistance anomaly signals first-order transition The key to detecting this transition in our study is the focused ion beam (FIB)-based fabrication of single crystal microstructures. This technique may become a powerful tool to detect subtle changes in the electronic matter of a wide range of materials ( Fig. 1b ). Details about device fabrication and an overview of the reproducibility of the results are given in the Methods section and in refs 18 , 19 . 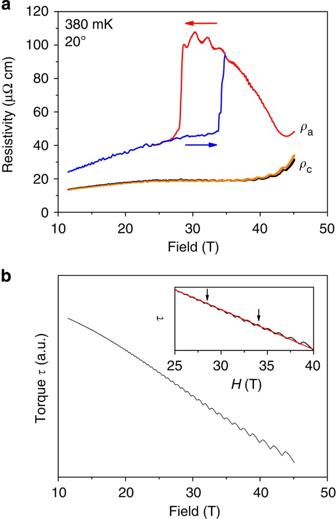Figure 2: Magnetoresistance and magnetic torque of CeRhIn5at 380 mK. Resistivity along thea- and thec-direction, as well as (b) the magnetic torque of CeRhIn5single crystals in fields tilted 20° away from thecaxis at 380 mK. The two main observations of this study become evident: a hysteretic, first-order-like transition in field occurring at ~30 T, which is marked by a salient jump in the in-plane resistivity. Remarkably, the out-of-plane resistivity, as well as the magnetic torque, remain featureless across the transition. The inset shows the torque on an amplified scale around the region of the resistive anomaly, with fields of the up- and downward resistivity jumps indicated by arrows and a linear fit to the data (red). Except for de Haas–van Alphen oscillations, the torque remains featureless in this region. This suggests a change in two-dimensional pieces of the Fermi surface prominent in the in-plane transport, but which do not contribute significantly to the out-of-plane transport. At the same time, the featureless torque indicates that a very subtle and practically imperceptible change in the magnetic susceptibility between the two states. Figure 2a shows the magnetoresistance ρ a (H) and ρ c (H) for currents flowing along both the in-plane and the inter-plane direction, respectively, at 380 mK for fields at an angle 20° away from the c axis. These traces immediately highlight the key observation of this study: the in-plane resistivity shows a step-like transition at 34 T to a high-resistive state (red), which more than doubles its value. This jump is followed by a region of negative magnetoresistance up to a minimum in resistivity at 42 T. On decreasing the magnetic field, the resistivity follows an upper hysteresis branch until it drops back onto the lower branch (blue) at 28 T. At the same time, the out-of-plane resistivity ρ c (H) remains featureless, indicating that mainly those electrons responsible for the in-plane transport participate in the transition. The magnetic torque τ = M × H was measured simultaneously with the transport samples using a capacitive cantilever technique ( Fig. 2b ). It shows pronounced de Haas–van Alphen oscillations, again highlighting the crystal quality, but otherwise remains featureless at the fields at which the jumps occur. Consequently, the Ce-4 f anti-ferromagnetic order remains unaffected and the transition occurs well within the AFM dome, in agreement with previous specific heat measurements [20] . Remarkably, the density of states at the Fermi level, therefore, does not change notably as often observed when the Fermi surface is reconstructed by a CDW or SDW. This indicates that the gapped Fermi surface sheet hosts comparatively light electrons, while the heavier sheets remain unaffected by the transition, which may be interpreted as a manifestation of the ‘two fluid’ description of heavy-fermion metals [21] . The contrasts between the subtle signs for a phase transition in the torque measurements on macroscopic crystals and the sharp features in the charge transport measurements on microstructures is remarkable. As multiple Fermi surface sheets with both two- and three-dimensional character are present in the material, the strong response of ρ a to the gapping of comparably few charge carriers suggests a large in-plane electron mobility of the gapped band. Figure 2: Magnetoresistance and magnetic torque of CeRhIn 5 at 380 mK. Resistivity along the a - and the c -direction, as well as ( b ) the magnetic torque of CeRhIn 5 single crystals in fields tilted 20° away from the c axis at 380 mK. The two main observations of this study become evident: a hysteretic, first-order-like transition in field occurring at ~30 T, which is marked by a salient jump in the in-plane resistivity. Remarkably, the out-of-plane resistivity, as well as the magnetic torque, remain featureless across the transition. The inset shows the torque on an amplified scale around the region of the resistive anomaly, with fields of the up- and downward resistivity jumps indicated by arrows and a linear fit to the data (red). Except for de Haas–van Alphen oscillations, the torque remains featureless in this region. This suggests a change in two-dimensional pieces of the Fermi surface prominent in the in-plane transport, but which do not contribute significantly to the out-of-plane transport. At the same time, the featureless torque indicates that a very subtle and practically imperceptible change in the magnetic susceptibility between the two states. Full size image Angular dependence of the critical field We have studied the angular dependence of the critical field H c by tilting the magnetic field in the ( a,c ) plane ( Fig. 3 ). The transition moves to higher field values as the field is rotated towards the a -direction. The upturn in angle does not follow a simple functional dependence; in particular, it does not behave as cos( θ ) −1 as one would expect if the out-of-plane field component would be the relevant parameter. Above angles of 60°, the transition becomes unobservable. This is accompanied by a gradual reduction of the relative amplitude of the resistive jump, that is, from its maximum at 20° to zero around 60°, indicating that at higher angles away from the c axis the charge order becomes energetically unfavourable. DWs in 3D metals arise due to a Fermi surface nesting enhancement of the susceptibility. One plausible scenario for a field-induced DW transition would be a progressive enhancement of Fermi surface nesting as the field deforms it in the presence of anisotropic and band-dependent g -factors. Such a mechanism would result in a highly non-trivial angular dependence for the critical magnetic field with respect to the crystallographic axes. The interaction between the f -electrons and the conduction electrons is known to give rise to Lifshitz transitions that change the Fermi surface topology by tuning a parameter such as pressure [22] or chemical substitution [23] . Yet, in contrast to the appearance of the DW, these transitions commonly involve a change in the anti-ferromagnetically ordered and localized 4 f states. 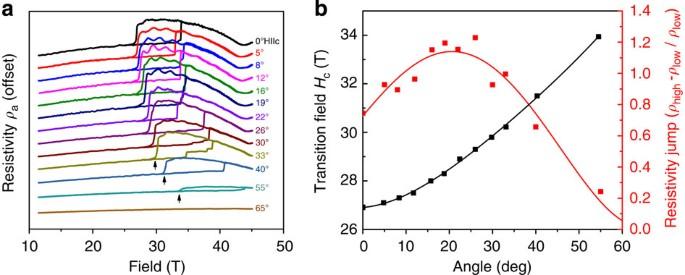Figure 3: Angular dependence. (a) In-plane resistivity as a function of the magnetic field at 380 mK, for various field angles relative to thecaxis, that is, from 0° (=H||c) to 65° as the field is rotated towards theb-direction. The field remained perpendicular to the applied current in a transverse magnetoresistance configuration at all studied angles. The drop at lower fields appears reproducibly at the transition fieldHcunder all experimental conditions. The position in field of the jump from the low resistance into the high-resistance state at higher fields, however, depends on external conditions such as the applied current, field sweep rate and angle. The largest hysteresis was obtained by using slow field sweep rates (1 T min−1) and low currents (400 μA). Nevertheless, jumps to intermediate resistivity values were observed, especially at higher angles. (b) Field position of the drop from the high- into the low-resistance state (Hc, marked by arrows in a), as well as the height of the drop relative to the low-resistivity branch. The lowest transition field is observed for fields along thecaxis, and the transition field increases on tilting the field towards theb-direction untilθ~60°, above which no transition is observable. The relative height of the drop is difficult to define with precision due to the resistance oscillations in the high-field state arising from the angle-dependent Shubnikov–de Haas effect. The relative drop is maximal at around 20° away fromcaxis and decays on further rotation of the field away from thecaxis, until the transition becomes undetectable at ~60°. Figure 3: Angular dependence. ( a ) In-plane resistivity as a function of the magnetic field at 380 mK, for various field angles relative to the c axis, that is, from 0° (=H|| c ) to 65° as the field is rotated towards the b -direction. The field remained perpendicular to the applied current in a transverse magnetoresistance configuration at all studied angles. The drop at lower fields appears reproducibly at the transition field H c under all experimental conditions. The position in field of the jump from the low resistance into the high-resistance state at higher fields, however, depends on external conditions such as the applied current, field sweep rate and angle. The largest hysteresis was obtained by using slow field sweep rates (1 T min −1 ) and low currents (400 μA). Nevertheless, jumps to intermediate resistivity values were observed, especially at higher angles. ( b ) Field position of the drop from the high- into the low-resistance state ( H c , marked by arrows in a), as well as the height of the drop relative to the low-resistivity branch. The lowest transition field is observed for fields along the c axis, and the transition field increases on tilting the field towards the b -direction until θ ~60°, above which no transition is observable. The relative height of the drop is difficult to define with precision due to the resistance oscillations in the high-field state arising from the angle-dependent Shubnikov–de Haas effect. The relative drop is maximal at around 20° away from c axis and decays on further rotation of the field away from the c axis, until the transition becomes undetectable at ~60°. Full size image Non-linear transport in the DW state We interpret our observation as evidence for a field-induced DW transition involving in-plane electrons, which does not significantly affect either the c axis resistivity or the magnetic torque. One of the hallmarks of DW phenomena is a pronouncedly non-linear conductivity associated with an additional conduction channel due to the sliding of the DW state in parallel to the remaining, un-gapped quasiparticles [8] , [24] . For a DW at small electric fields, Coulomb interactions pin the DW to crystal defects, and the remaining free quasiparticles constitute the only accessible conduction channel. The pinning potential can be overcome by the application of an electric field beyond a certain threshold value E c , leading to the sliding motion of the DW that contributes to the conductivity. At the critical magnetic field, we observe the onset of this type of non-linearity ( Fig. 4 ). The large hysteresis allows us to make a strong argument: by preparing the system in the lower (blue) and upper (red) branch, we can compare the differential resistance under the exact same conditions of field and temperature. This also allows us to exclude artifacts such as field-dependent contact resistances and self-heating, as these extrinsic sources of error would not depend on the hysteretic state of the sample. The non-linearity was observed in the whole experimentally accessible high-field region up to 45 T, indicating the persistence of the DWs above the hysteretic region. 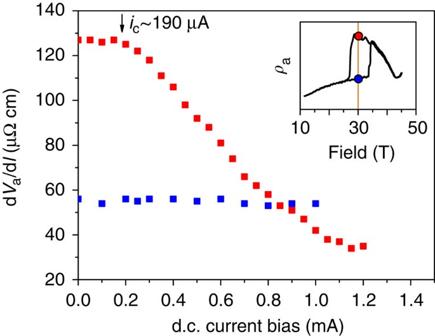Figure 4: Non-linear transport in the hysteretic region. The differential in-plane resistivity dVa/dI, measured by applying a small (10 μA r.m.s.) a.c. current superimposed onto a d.c. current bias, highlighting the key observation of this study. Both traces were measured under the same conditions at 30 T (20° away from thecaxis) and 380 mK. The system was prepared once in the low-resistance branch (blue), and then cycled to 45 T and back to reach the high-resistance branch (red). The zero-bias differential resistance changed by a factor of 2, indicating a successful state preparation. While in the low-resistivity branch the system remained ohmic over a wide range of current bias, the high-resistance branch shows pronouncedly non-linear transport. This behaviour is typical for pinned charge density waves, which are depinned by Coulomb forces exceeding the pinning force. Self-heating would not lead to a well-defined threshold electric field but rather to a parabolically increasing voltage response in contrast to what is seen. Figure 4: Non-linear transport in the hysteretic region. The differential in-plane resistivity d V a /d I , measured by applying a small (10 μA r.m.s.) a.c. current superimposed onto a d.c. current bias, highlighting the key observation of this study. Both traces were measured under the same conditions at 30 T (20° away from the c axis) and 380 mK. The system was prepared once in the low-resistance branch (blue), and then cycled to 45 T and back to reach the high-resistance branch (red). The zero-bias differential resistance changed by a factor of 2, indicating a successful state preparation. While in the low-resistivity branch the system remained ohmic over a wide range of current bias, the high-resistance branch shows pronouncedly non-linear transport. This behaviour is typical for pinned charge density waves, which are depinned by Coulomb forces exceeding the pinning force. Self-heating would not lead to a well-defined threshold electric field but rather to a parabolically increasing voltage response in contrast to what is seen. Full size image While the low-resistance branch (blue) remains ohmic up to high current densities, a pronouncedly non-linear differential resistance is observed in the upper branch (red). A well-defined critical current I c =190 μA separates the regions of pinned and sliding DW. Using the sample length l =34.6 μm and the low-current resistance R =280 mΩ in the upper branch, one finds a depinning-threshold electric field E c = RI c / l =15.2 mV cm −1 . Such E c of the order of 10 mV cm −1 are commonly observed in incommensurate CDW systems such as NbSe 3 and TaS 3 (refs 8 , 9 ). The large hysteresis presents us with the rare opportunity of studying a ‘supercooled’ electronic system and to compare the system with and without the DW under the same thermodynamic conditions. At the field-induced transition, the Fermi surface is reconstructed as indicated by a change in the Shubnikov–de Haas frequency spectrum ( Fig. 5 ). Besides a change in amplitude owing to the overall increase of the signal at the transition, two frequencies around 4,680 and 5,400 T appear in the high-field state, indicating the appearance of a new Fermi surface cross-section [25] . By using a smaller field window for the frequency analysis of the metastable region only ( Fig. 5 , middle), we can show that these frequencies are absent in the lower and present in the upper branch in the same field region. Since a reconstruction of the Fermi surface indicates the thermodynamic nature of the observed phase transition, the hysteretic appearance of this additional frequency firmly establishes it as a first-order phase transition. 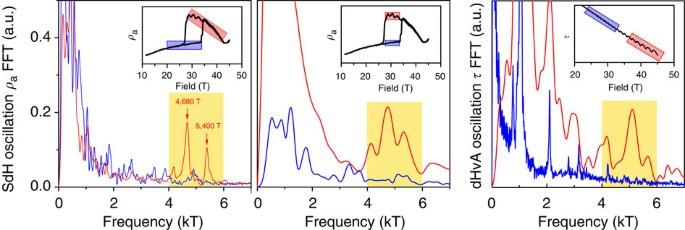Figure 5: Quantum oscillations indicate a Fermi surface reconstruction. Comparison between the Shubnikov–de Haas frequencies observed in the in-plane transport across the hysteretic transition (left), as well as de Haas–van Alphen oscillations measured by magnetic torque (right) for 20° away from H||c. On entering the high-resistance state (red), two new frequencies appear, and thus indicate a Fermi surface reconstruction at the transition. The large hysteresis allows to directly compare the frequency spectrum of the upper branch with the lower branch within the same field window (middle). The high-frequency oscillations appear over the whole hysteretic region on the upper branch and are completely absent in the lower branch. The appearance of the frequency can thus be clearly linked to the transition, and does not occur simply due to the enhancement of quantum oscillations in higher fields. The magnetic torque is a thermodynamic quantity, and can thus shed light on the thermodynamic character of the transition. We observe the appearance of high-frequency components also in the torque, in agreement with ref.28, indicating the thermodynamic nature of the transition despite the absence of a clear anomaly. Figure 5: Quantum oscillations indicate a Fermi surface reconstruction. Comparison between the Shubnikov–de Haas frequencies observed in the in-plane transport across the hysteretic transition (left), as well as de Haas–van Alphen oscillations measured by magnetic torque (right) for 20° away from H|| c . On entering the high-resistance state (red), two new frequencies appear, and thus indicate a Fermi surface reconstruction at the transition. The large hysteresis allows to directly compare the frequency spectrum of the upper branch with the lower branch within the same field window (middle). The high-frequency oscillations appear over the whole hysteretic region on the upper branch and are completely absent in the lower branch. The appearance of the frequency can thus be clearly linked to the transition, and does not occur simply due to the enhancement of quantum oscillations in higher fields. The magnetic torque is a thermodynamic quantity, and can thus shed light on the thermodynamic character of the transition. We observe the appearance of high-frequency components also in the torque, in agreement with ref. 28 , indicating the thermodynamic nature of the transition despite the absence of a clear anomaly. Full size image Interestingly, a low-frequency quantum oscillation is found to be strongly enhanced above the DW transition at smaller field angles ( Fig. 2 ). Its amplitude shrinks on increasing the magnetic field, contrary to the usual amplitude growth with field as described by the Lifshitz-Kosevich formalism [25] . One possible explanation for this unusual behaviour may be the proximity to the field-induced suppression of the AFM order at 50 T and the associated delocalization of the f -electrons. The onset of the AFM order at T N localizes the f -electrons and removes most of their spectral weight from the Fermi surface [26] . As the magnetic field suppresses the AFM, the f -electrons are expected to gradually delocalize, which leads to a field-dependent increase of the effective mass and thus to a suppression of the oscillatory amplitude at constant temperature. A similar enhancement of effective masses on approaching the AFM quantum critical point by pressure has been previously observed [27] . This anomalous reduction in amplitude may be related to the previously reported de Haas–van Alphen amplitude anomalies in CeRhIn 5 within this field and temperature range [28] . An important aspect of the observed DW is to what extent the order includes charge and spin degrees of freedom. Conventional incommensurate CDW and SDW lead to similar non-linear transport characteristics. While the experiment cannot unambiguously distinguish between these states, the experimental evidence seems more consistent with charge order. First of all, SDW-like anti-ferromagnetic transitions often yield pronounced changes in the anisotropic susceptibility χ (ref. 29 ), which were not detected by our magnetic torque measurements. The sample-size dependence of the hysteretic region presents another indication for a CDW-like state at high magnetic fields. A CDW arises from a coupling of the electronic system to the crystal lattice, and its appearance is accompanied by a lattice distortion. A sample of significantly larger dimensions ( Fig. 6 , width: 24 μm, thickness: 5.6 μm) was studied under the same conditions. In this larger sample, the hysteretic region is smaller and the transition is broadened compared with the step-like transition in the small sample. One plausible explanation would be a difference in strain relaxation in the two samples. As both microstructures are similarly coupled with the substrate, the elastic force of the mounting glue might impede a structural transition in the small sample while the large sample may more easily relax towards the new equilibrium. This would be in agreement with the observed change in the hysteresis and point towards a coupling of the order parameter to the lattice. 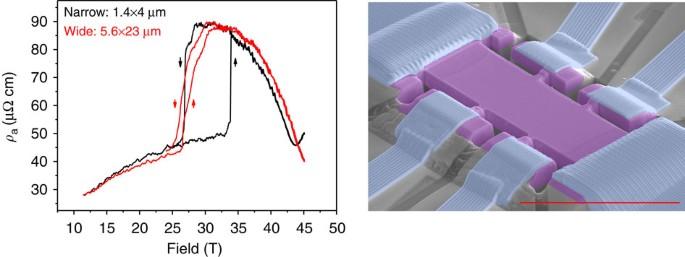Figure 6: Sample width dependence. In-plane resistivityρafor the small sample whose data are displayed throughout this study (seeFig. 1, black trace), as well asρafrom a larger device (red trace) shown on the right panel, both for fields aligned with thecaxis. The overall magnetoresistance behaviour agrees well among both samples; however, the hysteresis loop is significantly larger in the small sample. The DW transition for the large sample occurs at the same critical field as the one observed for the small sample when the field is swept down, thus indicating that this field of 27 T is closer to the thermodynamically relevant critical fieldHc. Scale bar, 50 μm. Figure 6: Sample width dependence. In-plane resistivity ρ a for the small sample whose data are displayed throughout this study (see Fig. 1 , black trace), as well as ρ a from a larger device (red trace) shown on the right panel, both for fields aligned with the c axis. The overall magnetoresistance behaviour agrees well among both samples; however, the hysteresis loop is significantly larger in the small sample. The DW transition for the large sample occurs at the same critical field as the one observed for the small sample when the field is swept down, thus indicating that this field of 27 T is closer to the thermodynamically relevant critical field H c . Scale bar, 50 μm. Full size image Yet, in the presence of strong magnetic fields, the nesting vector q will be field dependent due to the Zeeman-splitting of the Fermi surface and a pure CDW will become unstable in a similar way as a superconductor transitioning into an Fulde-Ferrell-Larkin-Ovchinnikov (FFLO) state. It was shown that in this situation an unconventional DW involving both charge and spin degrees of freedom may emerge as the new ground state at high magnetic fields [30] . Such an unconventional charge order has been observed in high magnetic fields in low-dimensional materials such as (Per) 2 Pt(mnt) 2 , which shows remarkable similarities to our findings [31] . Such DW instabilities are well understood in low-dimensional materials arising from the enhancement of the susceptibility on reducing the dimensionality [32] . Yet, CeRhIn 5 shows nearly isotropic transport properties in zero field ( Fig. 7 ), and further theoretical treatment will be required to understand this phenomenon in the context of low-dimensional Fermi surface sheets coexisting with strongly 3D sheets [10] in the presence of sizable magnetic fields. In addition, the driving force of this instability will have to be identified and the observation of a DW emphasizes the need to consider the often neglected role of electron–phonon coupling in heavy-fermion systems. Such coupling, however, is a natural consequence of the sensitivity of the ground state to small changes in bond lengths [2] . 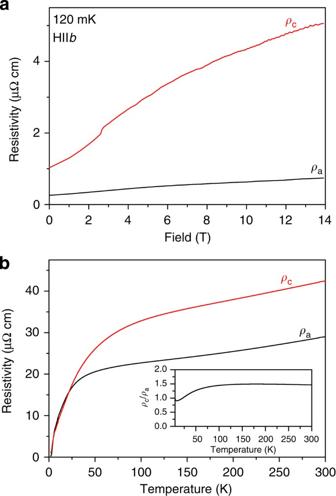Figure 7: Resistivity of the microstructured CeRhIn5devices. (a) Magnetoresistance along both crystallographic directions atT=100 mK and in fields up to 14 T. The Shubnikov–de Haas oscillations are sensitive to lowest levels of impurities, and their observation and agreement with bulk samples demonstrates the high crystal quality of the device. (b) Temperature dependence of the resistivity along both crystal directions in zero field. The temperature dependence matches quantitatively to previous measurements in bulk CeRhIn5crystals. The high residual resistivity ratio and the low resistivities achieved at low temperatures indicate the high quality of the studied devices. Inset: temperature dependence of the resistivity anisotropy. Figure 7: Resistivity of the microstructured CeRhIn 5 devices. ( a ) Magnetoresistance along both crystallographic directions at T =100 mK and in fields up to 14 T. The Shubnikov–de Haas oscillations are sensitive to lowest levels of impurities, and their observation and agreement with bulk samples demonstrates the high crystal quality of the device. ( b ) Temperature dependence of the resistivity along both crystal directions in zero field. The temperature dependence matches quantitatively to previous measurements in bulk CeRhIn 5 crystals. The high residual resistivity ratio and the low resistivities achieved at low temperatures indicate the high quality of the studied devices. Inset: temperature dependence of the resistivity anisotropy. Full size image Given the differences in the electronic structure between CeRhIn 5 and YBa 2 Cu 3 O 7−δ , the signatures of a high-field charge order in both systems share surprising similarities: there is no clear anomaly at the charge order transition in CeRhIn 5 observed in the torque measurements, contrary to conventional CDW materials such as NbSe 3 (ref. 33 ). It remains an open question as to why the CDW in YBa 2 Cu 3 O 7− δ can be well observed by NMR or X-ray diffraction experiments, yet heat capacity, resistivity or magnetic torque studies do not reveal any anomaly at the field-induced transition [34] . This may result from very small changes in entropy at the transition or be related to the intrinsic time constants of the different measurement techniques, and thus their different sensitivities to fluctuating order. It suggests that other experimental techniques such as high-field NMR should be performed in CeRhIn 5 , to clarify the so far unknown microscopic structure of the DW. The absence of a magnetization anomaly indicates that the field-induced charge-ordered state in both compounds is a similarly ‘subtle’ order, involving only a relatively small fraction of light carriers. This highlights a different aspect of the similarity between cuprates and Ce-based ‘115’ materials: Apparently, there is an almost undetectably small number of electrons in low-dimensional orbits present in both material classes that can drive a phase transition in moderately high magnetic fields perhaps involving the lattice degrees of freedom, yet without strong influence on the remaining carriers. FIB sample fabrication All presented devices were extracted from macroscopic (>3 mm) single crystals that were characterized by X-ray and checked for signs of indium impurities in a Superconducting Quantum Interference Device (SQUID). The single crystals were then analysed in a scanning electron microscope for surface defects. A clean, scratch-free part of the crystal was selected and the crystal was oriented using X-ray diffraction. In an initial step, a coarse ( a , c ) lamella with dimensions of ~60 × 60 × (7–8) μm 3 was carved out of the crystal bulk with a 2.5 nA, 30 kV Ga 2+ FIB (FEI Helios Nanolab 600i). The ( a , b ) face of the crystal was perpendicular to the ion beam during this process. In the next step, the sample was rotated in situ by 52°, to undercut the slice at 2.5 nA, 30 kV. In the last preparation step, the lamella was polished carefully using a lower current of 430 pA, 30 kV to remove potential damage layers from the high flux beam and to thin the lamella to its final thickness intended for the respective device (2–5 μm). The lamella was then transferred onto a Si chip with photolithographically prepared Au leads, connecting the final structure to bonding pads. The crystal slice was extracted ex situ and glued into the centre of this chip using a small amount of epoxy glue. In a final procedure, the sample was reintroduced into the FIB, for further carving and electric contacts. The sample was contacted with ion-assisted chemical vapor deposition (ia-CVD) deposited Pt in the FIB, at high ion flux to minimize resistance of the leads (2.5–9 nA, 30 kV). The typical resistance of each lead prepared this way was 20 Ω. In addition, the square platelet was further cut into the shape shown in the main Fig. 1 using low currents (430 pA, 30 kV). Preparing such a sample requires 4–5 full days of FIB work. This microstructuring procedure is essential for this experiment for four main reasons: The low resistivity of CeRhIn 5 leads to very small signals in typically milimetre-sized as-grown crystals at the low currents required to avoid self-heating at low temperatures. After microstructuring the crystal into a long (~30 μm) and thin (~5.5 μm 2 ) bar, the resistance is greatly enhanced by the geometrical factor, facilitating high-precision measurements in the challenging environment of strong magnetic fields. In addition, the FIB-deposited contacts were previously shown to perform reliably in pulsed-field conditions. While the zero-field resistivity at low temperatures is only moderately anisotropic, significant and field-dependent anisotropy develops in magnetic fields. Therefore, it is essential to ensure a homogeneous current profile in the sample to avoid field-dependent current redistribution due to changing anisotropy. The FIB microbars featuring side-contacts on a long bar are ideally suited to reliably distinguish between in- and out-of-plane resistivity. Furthermore, high current densities can be achieved in such devices by applying only moderate currents due to the micron-sized cross-section. While in principle low-resistance contacts could sustain similar current densities with some self-heating, currents of a few Ampere would not be feasible in high magnetic fields due to the extreme Lorentz force acting on the wires. As CeRhIn 5 is a good conductor, sustaining the depinning electric field E c requires a substantial current density that would be impractical in macroscopic crystals. In addition, in micron-sized samples, single domains may be isolated, allowing the study of intrinsic properties without the complications arising from domain dynamics. Reproducibility The FIB technique used to microstructure the single crystals of CeRhIn 5 studied here involves high-energy ion irradiation, and thus one has to take great care to investigate significant defects or changes to the material that may have been introduced by this preparation. We have found no sign of material degradation in any of the samples and in fact our current experimental evidence points towards a consistently high quality of such devices prepared out of heavy-fermion compounds. We observed consistently large residual resistivity ratios in all prepared devices well exceeding 200. The sample mainly used throughout this study showed residual ratios of ρ a (300 K)/ ρ a (80 mK)~258 and ρ c (300 K)/ ρ c (80 mK)~268. Another evidence for the high quality of our devices is the observation of Shubnikov–de Haas oscillations in fields as low as 4 T. This oscillatory phenomenon originates from the quantization of electronic orbits on the Fermi surface into Landau levels and is known to be exceptionally sensitive to defects ( ω c τ ~1-criterion) [25] . Its observation is generally accepted as strong evidence for very clean samples with a long mean-free path. This led us to conclude that the FIB process did not introduce significant scattering. Nine FIB-prepared samples of different shapes and sizes were produced and characterized in fields up to 14 T, and all of them have shown Shubnikov–de Haas oscillations. Particularly, the possibility of sample artifacts mimicking the reported DW transition was carefully checked. During the FIB process, some peculiar type of defect such as a microcrack could have been introduced into the sample, causing extrinsic physical parameters such as field and temperature to conspire in a way to artificially create the observed resistivity jump. This scenario is highly unlikely, as the jump is accompanied by changes of the Shubnikov–de Haas spectrum, which indicates the thermodynamic nature of the transition. To nonetheless exclude such extrinsic phenomena, a total of nine samples were prepared and four of them studied in high fields, in d.c. fields at the National High Magnetic Field Laboratory in Tallahassee (NHMFL), as well as in pulsed fields in the Pulsed Field Facility at Los Alamos National Laboratory (NHMFL-PFF). All studied samples consistently showed this transition at the same critical fields; however, no hysteresis was observed in pulsed fields, indicating the highly metastable character of the lower branch ( Fig. 8 ). At high ramp rates and high currents, the hysteresis also disappeared in d.c. fields as expected for metastability in first-order transitions. 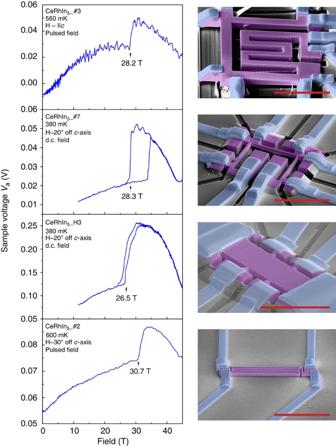Figure 8: Reproducibility. Various sample designs prepared to investigate the influence of the microstructure shape on the transition. Scale bars, 50 μm. Different types of sample designs from the U-shaped sample mainly shown in the manuscript, to thick and wide slabs, to thin, spring-like meander designs were fabricated. Two of them, CeRhIn5_#7 and CeRhIn5_H3 were mounted on epoxy glue, while the other two were not. These different types of mounting were used to check for the potential influence of strain originating from the differential thermal contraction. The consistent observation of Shubnikov–de Haas oscillations in the samples rules out significant strain, as inhomogeneous pressure smears out the frequencies and prevents their observation. All studied samples show the DW transition in quantitative agreement, regardless of the sample shape. Figure 8: Reproducibility. Various sample designs prepared to investigate the influence of the microstructure shape on the transition. Scale bars, 50 μm. Different types of sample designs from the U-shaped sample mainly shown in the manuscript, to thick and wide slabs, to thin, spring-like meander designs were fabricated. Two of them, CeRhIn 5 _#7 and CeRhIn 5 _H3 were mounted on epoxy glue, while the other two were not. These different types of mounting were used to check for the potential influence of strain originating from the differential thermal contraction. The consistent observation of Shubnikov–de Haas oscillations in the samples rules out significant strain, as inhomogeneous pressure smears out the frequencies and prevents their observation. All studied samples show the DW transition in quantitative agreement, regardless of the sample shape. Full size image How to cite this article: Moll, P. J. W. et al . Field-induced density wave in the heavy-fermion compound CeRhIn 5 . Nat. Commun. 6:6663 doi: 10.1038/ncomms7663 (2015).